High-energy spin and charge excitations in electron-doped copper oxide superconductors The evolution of electronic (spin and charge) excitations upon carrier doping is an extremely important issue in superconducting layered cuprates and the knowledge of its asymmetry between electron- and hole-dopings is still fragmentary. Here we combine X-ray and neutron inelastic scattering measurements to track the doping dependence of both spin and charge excitations in electron-doped materials. Copper L 3 resonant inelastic X-ray scattering spectra show that magnetic excitations shift to higher energy upon doping. Their dispersion becomes steeper near the magnetic zone centre and they deeply mix with charge excitations, indicating that electrons acquire a highly itinerant character in the doped metallic state. Moreover, above the magnetic excitations, an additional dispersing feature is observed near the Γ-point, and we ascribe it to particle-hole charge excitations. These properties are in stark contrast with the more localized spin excitations (paramagnons) recently observed in hole-doped compounds even at high doping levels. The differences and similarities between the electron- and hole-doped classes of superconductors have been one of the central subjects in the studies of the copper oxides [1] . Although the superconductivity shows up upon both electron and hole dopings, some anomalous physical properties, such as pseudogap and stripe orders, vary with the sign of the doped carriers. Therefore clarification of the differences and similarities is crucially important for understanding the emergence of high- T c superconductivity—and likewise of Mott insulator behavior—in strongly correlated electron systems, as it imposes constraints on the theoretical models. Extensive works for this purpose have been done since the discovery of the high- T c superconductivity and it is now established that carrier doping to the parent antiferromagnetic Mott insulator induces a metallic state, where the superconductivity in the cuprates emerges. Electrons in the metallic state often reveal both itinerant and localized characters, and the dual nature is a difficulty of the doped Mott insulators. It is generally believed that superconductivity in cuprates is intimately related to the antiferromagnetic spin fluctuation and inelastic neutron scattering (INS) has been widely used for studying the spin dynamics in the reciprocal lattice space. On the other hand, momentum-resolved excitation spectra of the charge degrees of freedom have been less explored because of the limitations of this experimental technique, even though both degrees of freedom should be clarified for the comprehensive understanding of cuprates. Magnetic excitations of the undoped parent compounds are fairly well described by spin-wave theory and the superexchange interaction between the nearest-neighbor Cu spins is found to be of the order of 100 meV (refs 2 , 3 , 4 ). Upon hole doping, the magnetic excitations change substantially and the ‘hour-glass’ dispersion appears [5] , [6] . Below the energy E cross at the waist of the hour-glass, the excitations disperse downward to the incommensurate wave vector away from the antiferromagnetic ordering vector q AF =(0.5,0.5) of the parent compounds. On the other hand, the dispersion of the excitations above E cross remains rather similar to that of the antiferromagnetic undoped compounds and a magnon-like mode survives. Very recently, resonant inelastic X-ray scattering (RIXS) at the Cu L 3 -edge has become an alternative to neutron scattering to measure momentum-resolved magnetic excitations [7] , [8] . RIXS complementarily covers the momentum space around the Γ-point, where high-energy magnetic excitations are hard to measure with INS, but cannot reach q AF . RIXS studies of the hole-doping dependence clarified that intense magnetic excitations remain as a paramagnon even in the overdoped region and its dispersion relation and energy-integrated spectral weight appear to be almost independent of the hole concentration [9] , [10] , [11] , [12] . It is argued from the result that the high-energy magnetic fluctuation is a vital source of the superconductivity [9] . Although high transition temperatures ( T c ) are realized in hole-doped superconductors, exceeding 90 K in some materials, the transition temperatures of electron-doped superconductors are limited below ~25 K. Magnetic excitations of the electron-doped cuprates differ from the hole-doped ones; they exhibit commensurate peaks centred at q AF at low energy [13] . Just a few INS works studying the high-energy magnetic excitations have been published and they have covered a restricted number of electron concentrations [14] , [15] and, due to the cross-section limitation, only in the vicinity of q AF . This shortcoming can be overcome in part by using modern spallation neutron sources like J-PARC, but another complementary technique is required to cover the wide energy and momentum ranges. RIXS at the Cu L 3 -edge perfectly matches these requirements. Here we use Cu L 3 edge RIXS and its complements, INS and Cu K-edge RIXS, for studying the electron-doping dependence of high-energy spin excitations and their counterpart, charge excitations, comprehensively. We chose Nd 2− x Ce x CuO 4 (NCCO) and Pr 1.40− x La 0.60 Ce x CuO 4 (PLCCO) for RIXS and INS measurements, respectively. This is because the Pr M 5 -edge is too close to the Cu L 3 -edge to perform RIXS experiment and the large magnetic moment of Nd hampers the measurement of magnetic INS. We will later show that magnon dispersions of the undoped materials ( x =0) are very similar to each other, which is why the NCCO data obtained with RIXS and the PLCCO INS data can be compared meaningfully. 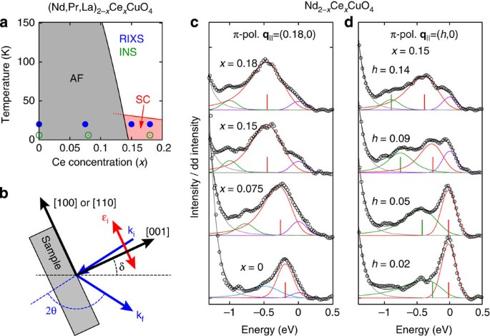Figure 1: Phase diagram and typical Cu L3-edge RIXS spectra. (a) Generic phase diagram of the electron-doped copper oxide superconductor (Nd,La,Pr)2−xCexCuO4. AF and SC denote antiferromagnetic and superconducting phases, respectively. Phase boundary of the superconductivity is slightly different between Nd2−xCexCuO4(x~0.14) and Pr1.40−xLa0.6CexCuO4(x~0.12). Filled and open circles indicate measured points of Cu L3-edge RIXS and INS, respectively. (b) Experimental configuration of Cu L3-edge RIXS. The scattering angle (2θ) is fixed at 130°.δis the rotation angle of the sample from specular toward grazing emission conditions. We takeq||>0 [h>0 inq||=(h,0) or (h,h)] forδ>0. (c,d) Cu L3-edge RIXS spectra of Nd2−xCexCuO4in the π-polarization conditions for (c) doping dependence at the fixed in-plane momentumq||=(0.18,0) and (d) momentum dependence ofx=0.15 near the Γ-point. The experimental spectra (open circles) are decomposed into a few components (solid lines). Peak positions of the spin-flip magnetic component (red) and charge excitations (green) are indicated by vertical bars. Detailed fitting procedure is described in Methods. Figure 1a shows a generic phase diagram of (Nd,Pr,La) 2− x Ce x CuO 4 as a function of the Ce concentration. We selected representative Ce concentrations for the present study: x =0 (undoped antiferromagnet), 0.075 (doped antiferromagnet), 0.15 (optimally doped superconductor) and 0.18 (overdoped superconductor) for NCCO and x =0, 0.08 and 0.18 for PLCCO. The temperature of the samples was, respectively, kept at 20 and 6 K for RIXS and INS, which are below the antiferromagnetic or superconducting transition temperature. Figure 1: Phase diagram and typical Cu L 3 -edge RIXS spectra. ( a ) Generic phase diagram of the electron-doped copper oxide superconductor (Nd,La,Pr) 2− x Ce x CuO 4 . AF and SC denote antiferromagnetic and superconducting phases, respectively. Phase boundary of the superconductivity is slightly different between Nd 2− x Ce x CuO 4 ( x ~0.14) and Pr 1.40− x La 0.6 Ce x CuO 4 ( x ~0.12). Filled and open circles indicate measured points of Cu L 3 -edge RIXS and INS, respectively. ( b ) Experimental configuration of Cu L 3 -edge RIXS. The scattering angle (2 θ ) is fixed at 130°. δ is the rotation angle of the sample from specular toward grazing emission conditions. We take q || >0 [ h >0 in q || =( h ,0) or ( h , h )] for δ >0. ( c , d ) Cu L 3 -edge RIXS spectra of Nd 2− x Ce x CuO 4 in the π-polarization conditions for ( c ) doping dependence at the fixed in-plane momentum q || =(0.18,0) and ( d ) momentum dependence of x =0.15 near the Γ-point. The experimental spectra (open circles) are decomposed into a few components (solid lines). Peak positions of the spin-flip magnetic component (red) and charge excitations (green) are indicated by vertical bars. Detailed fitting procedure is described in Methods. Full size image In the present study, we establish from Cu L 3 -edge RIXS and INS that the magnetic excitations of the copper oxides shift to higher energy in a wide momentum space upon electron doping. It indicates that electrons in the electron-doped copper oxides have itinerant character in their dynamics of the sub-eV range, which is marked contrast to the more localized paramagnon picture in the case of hole doping. Above the magnetic excitations, an additional dispersive feature is observed in the Cu L 3 -edge RIXS spectra near the Brillouin ZC. Its peak positions are found to follow the dispersion of the particle-hole charge excitations observed in the K-edge RIXS spectra and thereby the dispersive feature is ascribed to the same origin. Magnetic excitations in Cu L 3 -edge RIXS We start with Cu L 3 -edge RIXS. Because of the high two-dimensionality of the electronic properties, we discuss the momentum in the CuO 2 plane ( q || ) in the tetragonal notation ( a = b ~3.945 Å, c ~12.1 Å (ref. 16 )) by neglecting the variation of the momentum along the c *-axis. The experimental configuration ( q || >0 and π incident polarization), schematically presented in Fig. 1b , is chosen to give the largest spectral weight of the spin-flip transition within the d x2-y2 orbital as compared with the other channels (charge and lattice excitations) [7] . Experimental details are described in the Methods and Supplementary Information . Figure 1c shows the doping dependence at q || =(0.18,0). As demonstrated inref. [8] , the low-energy spectrum of the undoped compound ( x =0) can be univocally decomposed into the elastic (purple), single-magnon (red) and multi-magnon (cyan) components, and the single-magnon component is dominant. Upon electron doping, the spectral weight clearly moves to higher energy and the width of the peak broadens. Moreover, as typically shown for x =0.15 in Fig. 1d , we found an additional peak (green) near the Γ-point in the doped compounds. It probably has charge origin, as discussed later. In Fig. 2 , we summarize the momentum and doping dependence of the Cu L 3 -edge RIXS spectra of NCCO. The results for x =0 ( Fig. 2a ) are similar to those in the previous studies on undoped cuprates [4] , [8] , [9] . The spectra are decomposed into three components as in the Fig. 1c , and the elastic and spin-flip components are found to be resolution-limited. The observed momentum dependence of the single-magnon components follows the dispersion of the spin-wave of the antiferromagnetic square lattice. 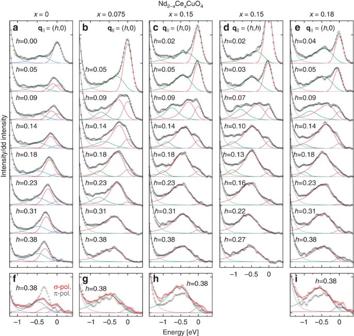Figure 2: Experimental data of Cu L3-edge RIXS. (a–e) Momentum dependence of the RIXS spectra of Nd2−xCexCuO4measured in π-polarization condition. Open circles are the experimental data and solid lines are the fitting results of elastic (purple), single-magnon (red), multi-magnon (cyan),ddexcitations at higher energy (grey) for the undoped compound, and sum of the all components (black). (a) In the doped compounds (b–e), we analyse the spectra using a single magnetic component (red) and an additional peak (green) at lowq||. Detailed fitting procedure is described in Methods. (f–i) Comparison of the spectra observed with incident σ and π polarization atδ=45°. Solid lines are the fitting results for σ-polarization. Figure 2: Experimental data of Cu L 3 -edge RIXS. ( a – e ) Momentum dependence of the RIXS spectra of Nd 2− x Ce x CuO 4 measured in π-polarization condition. Open circles are the experimental data and solid lines are the fitting results of elastic (purple), single-magnon (red), multi-magnon (cyan), dd excitations at higher energy (grey) for the undoped compound, and sum of the all components (black). ( a ) In the doped compounds ( b – e ), we analyse the spectra using a single magnetic component (red) and an additional peak (green) at low q || . Detailed fitting procedure is described in Methods. ( f – i ) Comparison of the spectra observed with incident σ and π polarization at δ =45°. Solid lines are the fitting results for σ-polarization. Full size image The spectra of the doped compounds in Fig. 2b–e cannot be decomposed in the same way as the undoped ones in Fig. 2a because of the intrinsic broadening of the peaks. We analyse the spectra of the doped compounds for large q || by a single inelastic component, which has been adopted from the published works of the hole-doped compounds. The main portion of the spectral weight is assigned to the spin-flip excitations [9] , [10] , [11] , [12] . This assignment is supported by a recent theoretical study which demonstrates that the RIXS spectra of the π-incident polarization agree well with the dynamical spin correlation function, S ( q ,ω), even without outgoing polarization analysis [17] . In addition, the two-magnon component observed by Raman scattering is weakened by electron doping [18] , and it is therefore acceptable to neglect the two-magnon component in the analysis of the doped compounds. As inelastic component, we use an antisymmetrized Lorentzian function convoluted by the Gaussian resolution. Details of the fitting analysis are described in Methods. The peak position and width obtained from the fittings are plotted against the momentum in Fig. 3a,b , respectively. We also plot the single-magnon components of the undoped compounds. Our RIXS results clearly demonstrate that the magnetic excitations shift to higher energy and broaden upon electron doping. It is notable that the high-energy shift of the magnetic excitation upon electron doping is consistent with a recent theoretical calculation [17] . 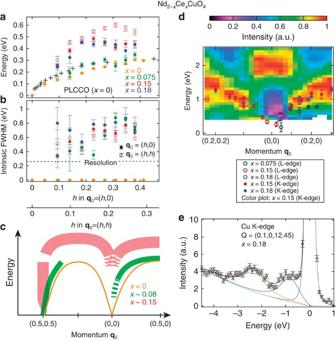Figure 3: Summary of magnetic and charge excitations. (a,b) Peak position and intrinsic width (full width at half maximum) of magnetic excitations. We plot the single-magnon component for the undoped compound (x=0). Peak positions of INS of undoped PLCCO are also shown by the crosses. The peak width of undoped NCCO (x=0) is fixed to infinitesimal in the analysis. The vertical bars represent the error in the fitting analysis. (c) Schematic of magnetic excitations in the energy-momentum space. (d) Peak positions of the additional peak feature above the magnetic excitations observed with Cu L3-edge (open circles). The background colour plot is the intensity map of the K-edge RIXS which is re-plotted from the data in ref.22. We also plot the peak position of the K-edge RIXS forx=0.15 and 0.18 (filled circles). Vertical bars on the plotted circles indrepresent the error in the fitting analysis inFigure 2. (e) Cu K-edge RIXS spectrum of NCCO (x=0.18). The spectrum is decomposed into elastic (purple), intraband (green) and interband (yellow) excitations, and the tail of high-energy excitation (grey). Error bars are determined by counting statistics. Figure 3: Summary of magnetic and charge excitations. ( a , b ) Peak position and intrinsic width (full width at half maximum) of magnetic excitations. We plot the single-magnon component for the undoped compound ( x =0). Peak positions of INS of undoped PLCCO are also shown by the crosses. The peak width of undoped NCCO ( x =0) is fixed to infinitesimal in the analysis. The vertical bars represent the error in the fitting analysis. ( c ) Schematic of magnetic excitations in the energy-momentum space. ( d ) Peak positions of the additional peak feature above the magnetic excitations observed with Cu L 3 -edge (open circles). The background colour plot is the intensity map of the K-edge RIXS which is re-plotted from the data in ref. 22 . We also plot the peak position of the K-edge RIXS for x =0.15 and 0.18 (filled circles). Vertical bars on the plotted circles in d represent the error in the fitting analysis in Figure 2 . ( e ) Cu K-edge RIXS spectrum of NCCO ( x =0.18). The spectrum is decomposed into elastic (purple), intraband (green) and interband (yellow) excitations, and the tail of high-energy excitation (grey). Error bars are determined by counting statistics. Full size image Magnetic excitations in INS While the electron-doping dependence in a large portion of the momentum space around the Γ-point is unveiled by the Cu L 3 -edge RIXS, INS can cover the momentum space near q AF . 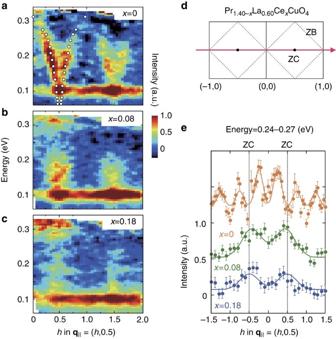Figure 4: Magnetic INS of PLCCO. (a–c) The momentum isq||=(h,0.5). The neutron scattering intensity normalized to the sample volume after subtracting the non-magnetic background at (0.8, 0.2) is multiplied by ω2to exhibit the entire spectrum with emphasizing the high-energy intensity. Open circles inaare the peak positions of magnon excitations. Dispersionless crystal field excitations of Pr are overlapped around 100, 320 meV. (d) Reciprocal lattice of the CuO2plane. ZC and ZB are the magnetic zone centre and zone boundary, respectively. The abscissa of the figures (a–c,e) follows the arrow. (e) Constant energy cut of INS intensity maps. Data are shifted vertically for clarity. To see the peak-shift upon doping, each data set was fitted by Gaussian functions. The solid lines are the best fitted result. The error bars ineindicate the statistical error (s.d. to the number of detected neutrons). They are determined by counting statistics. Figure 4a–c show magnetic INS spectra of PLCCO. For x =0 the spin-wave dispersion, indicated by the open circles in Fig. 4a , closely traces that of NCCO ( x =0) as obtained by RIXS: in Fig. 3a the INS data of undoped PLCCO is represented by the black crosses. When electrons are doped, the spectral weight at 100–300 meV accumulates gradually at q AF and it stands steeply at q || = q AF . Such a doping effect is clearer in the constant energy cut in Fig. 4e , where INS intensity at 240–270 meV is plotted as a function of momentum transfer. While the peak appears at the middle of the Brillouin zone in x =0, it remains at the magnetic zone centre (ZC) in x =0.18. In other words, the spectral weight at a certain momentum away from q AF moves toward higher energy upon doping, consistently with the Cu L 3 -edge RIXS results around the Γ-point. A detailed analysis of the INS results on PLCCO will be published elsewhere. Such spin excitations have been reported in electron-doped Pr 1- x LaCe x CuO 4 below 180 meV (refs 15 , 19 ), and the present study confirmed that they extend up to 300 meV. Alternatively, an analysis based on a two-dimensional spin-wave dispersion gave a larger nearest-neighbor coupling for Pr 1− x LaCe x CuO 4 ( x =0.12) than that for Pr 2 CuO 4 (ref. 14 ). It is noted that low-energy excitations (<15 meV) behave oppositely; the magnetic peak centred at q AF becomes broader in the momentum direction upon electron doping [20] , [21] . In Fig. 3c , we schematically summarize the magnetic excitation dispersion obtained by RIXS and INS. Figure 4: Magnetic INS of PLCCO. ( a – c ) The momentum is q || =( h ,0.5). The neutron scattering intensity normalized to the sample volume after subtracting the non-magnetic background at (0.8, 0.2) is multiplied by ω 2 to exhibit the entire spectrum with emphasizing the high-energy intensity. Open circles in a are the peak positions of magnon excitations. Dispersionless crystal field excitations of Pr are overlapped around 100, 320 meV. ( d ) Reciprocal lattice of the CuO 2 plane. ZC and ZB are the magnetic zone centre and zone boundary, respectively. The abscissa of the figures ( a – c , e ) follows the arrow. ( e ) Constant energy cut of INS intensity maps. Data are shifted vertically for clarity. To see the peak-shift upon doping, each data set was fitted by Gaussian functions. The solid lines are the best fitted result. The error bars in e indicate the statistical error (s.d. to the number of detected neutrons). They are determined by counting statistics. Full size image Charge excitations Now we turn to the additional peak (green in Fig. 1d ) above the magnetic excitation observed with Cu L 3 -edge RIXS. In Fig. 3d , we plot the peak positions of NCCO ( x =0.075, 0.15 and 0.18) obtain by the fitting analysis of the Cu L 3 -edge RIXS (green lines in Fig. 2b–e ) on the intensity map of the Cu K-edge RIXS re-plotted fromref. [22] . As spin-flip transitions are forbidden in K-edge RIXS, the intensity around 1–2 eV can be assigned only to charge excitations. Thus the dispersive features with momentum-dependent width are ascribed to intraband charge excitations (incoherent particle-hole excitations) within the upper Hubbard band, whereas interband excitations across the charge transfer gap are concentrated around 2 eV near the ZC [22] , [23] . The peak positions in the Cu L 3 -edge RIXS smoothly connect to the dispersive features in the Cu K-edge RIXS. In Fig. 3e , we show a K-edge RIXS spectrum of NCCO ( x =0.18), which was measured recently with better energy resolution than that inref. [22] . Both intraband and interband transitions are observed on the tail of an excitation at higher energy, and the peak position of the former agrees with that at q || =(0.09,0) in the Cu L 3 -edge RIXS of the same compound. Therefore, it seems reasonable to ascribe the additional excitation in the Cu L 3 -edge RIXS to the same charge origin as the dispersive mode in the K-edge RIXS, and it is possibly particle-hole excitations within the upper Hubbard band. The existence of the particle-hole excitations has been established in the t - J or Hubbard models (see Fig. 5 and Methods). The energy of particle-hole excitation is of the order of the transfer energy ( t ~400 meV), and it should be higher than the magnetic excitations at the energy scale of the exchange interaction ( J ~100 meV) in the models, which agrees with our assignment. Plasmon excitations might be another possible origin of the additional excitation in the Cu L 3 -edge RIXS. A theoretical work proposed that RIXS can probe dispersive plasmon excitations whose energy gap at the Γ-point depends on the out-of-plane momentum ( q z ) [24] . However solid assignment of the plasmon excitations in the experimental RIXS spectra has not been done so far. It may be tested by detailed dependence on q z . 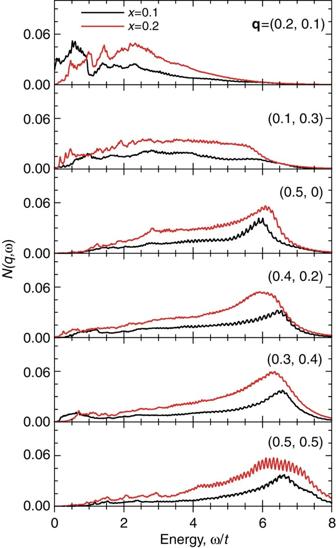Figure 5: Calculated dynamical charge correlation functionN(q,ω). The dynamical charge correlation function is calculated for an electron-dopedN=20t-t'-t''-Jlattice with three-site terms. Averaging over twisted boundary condition is applied. Black and red curves correspond to the carrier concentration ofx=0.1 and 0.2, respectively. Figure 5: Calculated dynamical charge correlation function N (q,ω). The dynamical charge correlation function is calculated for an electron-doped N =20 t-t'-t''-J lattice with three-site terms. Averaging over twisted boundary condition is applied. Black and red curves correspond to the carrier concentration of x =0.1 and 0.2, respectively. Full size image The doping evolution of the charge excitations is momentum-dependent. At the low-| q || | region, the spectral weight of the charge excitations shifts to higher energy with increasing electron concentration, which is evidenced by the Cu L-edge RIXS in Fig. 3d . On the other hand, the spectral weight increases almost at the same energy with doping at high | q || | and high energy, for example, h ≥0.25 for q || =( h ,0) and above 1 eV. The latter has been confirmed by the K-edge RIXS [22] , [25] . This doping evolution is reproduced in the theoretical calculation of the dynamical charge correlation function, N ( q ,ω), shown in Fig. 5 . At the smallest q defined in the system of the calculation ( q =(0.2,0.1)), the spectral weight below ω~ t is larger than that in high-energy region near ω~2 t for x =0.1. Note that the low-energy weight is governed by the charge motion scaled by J due to spin-charge coupling, while the high-energy weight is caused by an incoherent motion of charge scaled by t (ref. 26 ). With increasing x , the low-energy weight is suppressed accompanied with the increase of the incoherent weight, leading to the shift of peak position to higher-energy region. Such a shift is consistent with the observed data shown in Fig. 3d . For larger value of q , the incoherent charge motion dominates the spectral weight independent of x . From the Cu L 3 -edge RIXS, complemented by INS and Cu K-edge RIXS, we have thus clarified the doping evolution of the spin and charge excitations in the electron-doped copper oxide superconductors. Notably, the spin-wave magnetic excitations of the undoped insulator shift to higher energy upon electron doping over a wide momentum space. This is in distinct contrast to the hole-doped case, where spectral distribution of the magnetic excitations broadens but keeps its energy position almost unchanged upon doping, namely, it follows rather closely the spin-waves dispersion of the parent compound [9] , [10] , [11] , [12] . It means that, in hole-doped copper oxides, the spin excitation at high energy is a remnant mode of the parent antiferromagnetic insulator and the spin dynamics has localized nature. On the other hand, the spectra reported in the present study reflect the strongly itinerant character of the electron-doped copper oxides. Actually, it was pointed out inref. [15] that the high-energy excitations around q AF in INS of PLCCO bear a close similarity of the spin excitations in the nearly antiferromagnetic metals, vanadium-doped Cr [27] and iron-doped Mn 3 Si [28] . The itinerant character of electron-doped compounds can be observed also by exploiting the polarization dependence of Cu L 3 -edge RIXS. It is known that at large positive values of q || , spin-flip magnetic excitations dominate in the π-polarization condition whereas they are negligible in the σ-polarization condition [7] , [29] . At δ =45°, the ratios of spin-flip ( d x2-y2 ↓→ d x2-y2 ↑) to spin-conserved ( d x2-y2 ↓→ d x2-y2 ↓) cross sections in the Cu 2+ single-ion model are 2.14 and 0.03 for π- and σ-polarizations, respectively. In Fig. 2f–i , we systematically compare the RIXS spectra measured with π- and σ-polarizations of incident photons. In the undoped compound ( Fig. 2f ), the single-magnon is clearly enhanced with π-polarization, as previously observed in other parent antiferromagnetic compounds [9] , [30] , and multi-magnon excitations make a dominant contribution to the σ-polarization spectrum. Such single-magnon dominance in the polarization dependence seems to persist for x =0.075, although to a lesser extent with respect to the hole-doped case [9] . When further increasing the electron concentration, the spectral shape becomes similar between the two polarizations; more precisely, the spectrum of the π-polarization is overlaid with that of the σ-polarization with its peak centre located at slightly higher energy. This means that in optimal and over-doped compounds magnetic (spin-flip) excitations mix with the charge (spin-conserved) excitations in the same energy scale. Probably, the σ-polarization spectra are mainly given by a continuum of electron-hole pair excitations and, in the same energy range, the spin-flip channel can be considered as sort of Stoner excitations: the almost flat dispersion far from q || =(0,0) and (0.5,0.5) may be an indication of the particle-hole-like nature of magnetic excitations. Therefore the electron dynamics of the electron-doped cuprates has highly itinerant character in the sub-eV energy scale, and the concept of paramagnon, which is valid up to the overdoped region in the hole-doping case [11] , [12] , does not work any more. Sample preparation We prepared Nd 2− x Ce x CuO 4 (NCCO) for RIXS and Pr 1.40− x La 0.60 Ce x CuO 4 (PLCCO) for INS. Single crystals of NCCO ( x =0, 0.075, 0.15 and 0.18) and PLCCO ( x =0, 0.08 and 0.18) were grown by the traveling-solvent floating-zone method. Doped NCCO crystals were annealed at 900 °C for 10 h in the Ar gas atmosphere. The Néel temperatures determined by elastic neutron scattering measurements for NCCO ( x =0, 0.075, 0.15 and 0.18) and PLCCO ( x =0, 0.08 and 0.18) were (269(5), 218(5), 63(18) and 10(5) K) and (278(8), 228(5) and 155(18) K). Superconducting transition temperatures of NCCO ( x =0.15 and 0.18) were (25(1) and 22(1) K). Cu L 3 -edge RIXS The Cu L-edge RIXS experiments were performed at beam line ID08 of the ESRF using the AXES spectrometer with linearly polarized x rays, either perpendicular (σ) or parallel (π) to the scattering plane. Total energy resolution was 250 meV. It is sufficient for the present study because most of the spectral features in the RIXS spectra are intrinsically broader than the energy resolution, as shown for the magnetic excitations in Fig. 3b . Incidentally we note that the instrument and the energy resolution used for this work are exactly the same as the work on doping dependence of the magnetic excitations in hole-doped La 2− x Sr x CuO 4 (ref. 12 ). The NCCO crystals were cleaved in the air and mounted on the spectrometer. The surface of the crystal was normal to the c axis, which was kept in the scattering plane so as to be scanned in the reciprocal lattice space spanned by either the [100]-[001] or the [110]-[001] axes. The experimental configuration is schematically presented in Fig. 1b of the main text. Momentum in the CuO 2 plane ( q || ) is changed by rotating the sample. In the present study, we scanned in the range of 0°≤| δ |≤45° and it corresponds to the reciprocal lattice space of 0≤| h |≤0.38 and 0≤| h |≤0.27 for q || =( h ,0) and q || =( h , h ), respectively. Temperature of the sample was kept at 20 K. We fit the RIXS spectra in the Figs 1c,d and 2 as follows. The elastic peak (purple line in the figures) is fit with a resolution-limited Gaussian function. The component of the spin-flip magnetic excitations (red) is modelled by an antisymmetrized Lorentzian function multiplied by the Bose factor and it is convoluted by the Gaussian resolution function. The width of the Lorentzian function is infinitesimal for the spectra of the undoped compound ( x =0) whereas it is variable for the doped compounds. The multi-magnon (cyan) and charge excitations (green) are also assumed by the antisymmetrized Lorentzian function. We include the tail of the dd excitations (grey) in the analysis. Because the decomposition of the elastic and magnetic components is difficult at very low | q || | ( h ≤0.05 for q || =( h ,0) and h ≤0.03 for q || =( h , h )) of the doped compounds, we do not include the elastic component for the analysis. Therefore we rely on INS for the peak positions of the magnetic component near the ZC. In the analysis of doped compounds, we include the charge excitations unless the spectral shape can be reproduced by the magnetic component (plus elastic scattering and dd excitations) alone. Then, the cut-off momenta for including the charge excitations are q || =(0.23,0) for x =0.075, q || =(0.18,0) and (0.13,0.13) for x =0.15, and q || =(0.18,0) for x =0.18. The charge excitations should exist above the cut-off momenta, but they are overlaid with the huge tail of dd excitations, which makes it difficult to evaluate the spectral weight of the charge excitations. Cu K-edge RIXS The Cu K-edge RIXS experiments of NCCO ( x =0.18) were carried out at BL11XU of SPring-8. A channel-cut Si(333) monochromator and a Ge(733) analyser were used and total energy resolution was 250 meV. The surface of the crystal was normal to the c axis and the a and c axes were kept in the horizontal scattering plane. Temperature of the sample was 20 K. INS INS spectra were measured by a direct-geometry chopper spectrometer 4SEASONS installed in the Materials and Life Science Experimental Facility in the Japan Proton Accelerator Research Complex (J-PARC). To cover a spin excitation in a wide energy range, the neutron incident energy of 357 meV was selected (half-width at half-maximum energy resolution of ~20 meV at the elastic position). The crystals were co-aligned so that the crystallographic c axis is parallel to the incident neutron beam. The total weight of PLCCO with x =0, 0.08 and 0.18 was 42.2, 42.6 and 28.1 g, respectively. For all samples, the temperature was controlled to be 6 K by a closed cycle refrigerator. Calculation of dynamical charge correlation function The dynamical charge correlation function was calculated for the t-t′-t″'-J model with three-site term. The Hamiltonian is given by with and where the summations , and run over first, second, and third nearest-neighbour pairs, respectively. The operator annihilates a localized particle with spin σ at site i with the constraint of no double occupancy, and S i is the spin operator at site i . In the model, we set t =1, t′ =−0.25, and t″ =0.12, and J =0.4 for electron doping. The real value of t in cuprates is usually taken to be 0.35 eV. The dynamical charge correlation function is defined as where is the ground state with energy E 0 and with number of site N and the position vector R i at site i . The small positive number γ is set to be 0.02 in our calculation. The doping dependence of N ( q ,ω) for a N =20 system is shown in Fig. 5 , where x =0.1 ( x =0.2) corresponds to the case of 2 (4) electrons in the system. An averaging procedure for twisted boundary conditions is used to reduce the finite-size effect [31] . How to cite this article: Ishii, K. et al. High-energy spin and charge excitations in electron-doped copper oxide superconductors. Nat. Commun. 5:3714 doi: 10.1038/ncomms4714 (2014).